Activation and splitting of carbon dioxide on the surface of an inorganic electride material Activation of carbon dioxide is the most important step in its conversion into valuable chemicals. Surfaces of stable oxide with a low work function may be promising for this purpose. Here we report that the surfaces of the inorganic electride [Ca 24 Al 28 O 64 ] 4+ ( e − ) 4 activate and split carbon dioxide at room temperature. This behaviour is attributed to a high concentration of localized electrons in the near-surface region and a corrugation of the surface that can trap oxygen atoms and strained carbon monoxide and carbon dioxide molecules. The [Ca 24 Al 28 O 64 ] 4+ ( e − ) 4 surface exposed to carbon dioxide is studied using temperature-programmed desorption, and spectroscopic methods. The results of these measurements, corroborated with ab initio simulations, show that both carbon monoxide and carbon dioxide adsorb on the [Ca 24 Al 28 O 64 ] 4+ ( e − ) 4 surface at RT and above and adopt unusual configurations that result in desorption of molecular carbon monoxide and atomic oxygen upon heating. Efficient and inexpensive conversion of CO 2 into valuable chemicals would simultaneously contribute to reducing CO 2 emission into the atmosphere and lessen the dependence of society on fossil fuels [1] , [2] . Activation and splitting of the CO 2 molecule are the most important steps in this process. However, because CO 2 is nonpolar and has two double bonds, its activation requires high temperature/pressure conditions and/or active reductants, such as hydrogen. Alternatively, CO 2 can be activated under ambient conditions with the help of a solid-state catalyst, the role of which is to adsorb CO 2 molecules and facilitate electron transfer to them [3] . Solid-state bases, such as alkaline earth metals and alkaline earth metal oxides, are known to be CO 2 sorbants, and numerous studies on the formation of ‘bent’ CO 2 δ − configurations on their surfaces have been reported [4] , [5] , [6] , [7] , [8] , [9] . However, formation of these CO 2 δ − species alone does not lead to CO 2 splitting. Surfaces of transition and sp metals, either on their own, such as Cu [10] , or doped with alkali metal atoms so as to reduce their work function, can activate CO 2 and generate CO through decomposition of CO 2 δ − and/or CO 3 δ − intermediates [11] , [12] , [13] . However, this approach is impractical for industrial applications because it requires a combination of low temperatures, delicate surface control and/or expensive metals. Thus, there is a need for new materials, which offer both high chemical stability and high ability to facilitate electron transfer to CO 2 and induce its dissociation. [Ca 24 Al 28 O 64 ] 4+ ( e − ) 4 , or C12A7: e − for brevity [14] , [15] , [16] , is an electride [17] , [18] , [19] , that is, a material in which electrons serve as anions. As shown in Fig. 1 , the crystal framework of C12A7: e − is formed by a three-dimensional network of interconnected cages with the inner diameter of ~0.4 nm. The cages each bear a positive charge of +1/3, which is compensated by extra-framework electrons—‘anionic electrons’—clathrated in them. The local atomic environment of these anionic electrons, in particular the arrangement of the nearest six Ca 2+ ions, is similar to that of an F + -centre in a CaO crystal, that is, an electron trapped at the site of an O 2− vacancy. The concentrations of the cages (~6 × 10 21 cm −3 ) and of the anionic electrons (~2 × 10 21 cm −3 ) in C12A7: e − are large enough to form a partially occupied band rather than a set of discrete energy levels. As the average cage diameter is ~1.5 times that of the oxygen vacancy in CaO and the cage wall charge is lower than that provided by the F + -centre environment, the Madelung potential at the cage centre is rather small. This explains why the work function of C12A7: e − is only 2.4 eV, which is close to that of potassium metal [20] . Furthermore, the anionic electrons confined to cages act as chemically active centres facilitating adsorption of molecular contaminants, such as H 2 O, O 2 and CO 2 , at the surface. However, the small size of the openings between the cages does not allow for these species to penetrate through the cage wall under ambient conditions. Thus, C12A7: e − is chemically inert despite its work function being comparable to that of highly reactive metals, such as alkali metals. 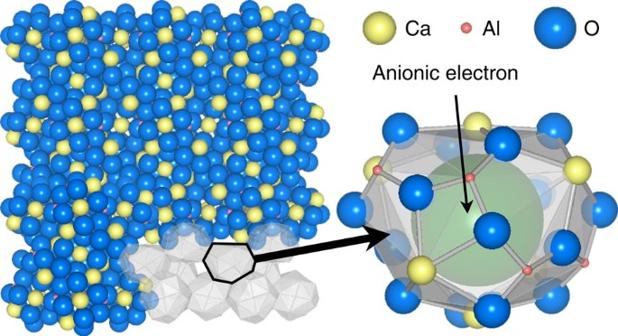Figure 1: Schematic illustration of the (100) surface of C12A7:e−. The model draws upon STM studies of C12A7:e−22. Yellow, red and blue spheres represent Ca, Al and O atoms, respectively. The lower right portion of the model is drawn without atom spheres, and the white polygons represent the interior spaces of the cages. The figure on the right shows magnification of the cages and the clathrated anionic electron (green sphere). Figure 1: Schematic illustration of the (100) surface of C12A7: e − . The model draws upon STM studies of C12A7: e − [22] . Yellow, red and blue spheres represent Ca, Al and O atoms, respectively. The lower right portion of the model is drawn without atom spheres, and the white polygons represent the interior spaces of the cages. The figure on the right shows magnification of the cages and the clathrated anionic electron (green sphere). Full size image In this article, we report that CO 2 adsorbed on the C12A7: e − surface dissociates into CO and atomic oxygen at room temperature (RT). Temperature-programmed desorption (TPD) measurements were carried out to estimate the capacity of the C12A7: e − surface to adsorb CO 2 . The adsorbed CO 2 and the products of its decomposition were analysed by photoelectron spectroscopy (PES) and Fourier transform infrared reflection absorption spectroscopy (FTIR-RAS). These experimental data, together with ab initio simulations, allowed us to establish the atomic-scale mechanism for adsorption and dissociation of CO 2 on the C12A7: e − surface. CO and CO 2 species on the surface of C12A7: e − To investigate whether CO 2 is adsorbed on the C12A7: e − surface, we compared the TPD spectra for several surfaces exposed to the same amount of C 18 O 2 (95% 18 O isotopic purity Isotech gas was used to eliminate the contribution of residual gases, such as C 16 O 2 and C 16 O). The data in Fig. 2a demonstrate that the TPD yield for C12A7: e − is noticeably larger than that for other oxide surfaces. 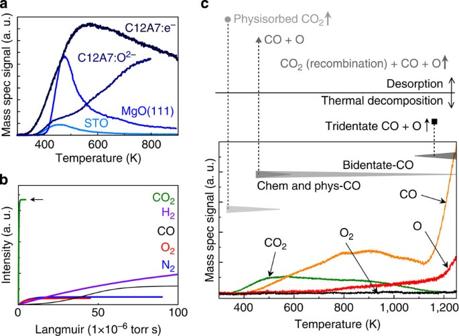Figure 2: TPD curves. (a) CO2(C18O2) TPD curves of C12A7:e−, C12A7:O2−(film), MgO (111) (film) and SrTiO3:Nb after 1 L of CO2exposure. (b) Saturation curves of CO2, H2, N2, O2and CO adsorption on the C12A7:e−surface. The curves were derived from the change in the degree of vacuum during TPD and the integrated areas under the TPD curves. (c) TPD curves of all desorption products from the C12A7:e−surface after 2 L of exposure to CO2at RT with the proposed CO2desorption and decomposition sequence. The intensities of the curves were calibrated by sensitivity factors. The heating rate was 0.5 K s−1. Figure 2b shows that adsorption of CO 2 reaches saturation at much lower exposure (~2 L) than in the case for H 2 , N 2 , O 2 and CO. Thus, these results demonstrate that C12A7: e − adsorbs CO 2 quickly and in large quantities compared with other gaseous species. We estimate the amount of adsorbed CO 2 to be at least 10 13 cm −2 , which agrees well with the density of anionic electrons at the C12A7: e − surface. Figure 2: TPD curves. ( a ) CO 2 (C 18 O 2 ) TPD curves of C12A7: e − , C12A7:O 2− (film), MgO (111) (film) and SrTiO 3 :Nb after 1 L of CO 2 exposure. ( b ) Saturation curves of CO 2 , H 2 , N 2 , O 2 and CO adsorption on the C12A7: e − surface. The curves were derived from the change in the degree of vacuum during TPD and the integrated areas under the TPD curves. ( c ) TPD curves of all desorption products from the C12A7: e − surface after 2 L of exposure to CO 2 at RT with the proposed CO 2 desorption and decomposition sequence. The intensities of the curves were calibrated by sensitivity factors. The heating rate was 0.5 K s −1 . Full size image TPD spectra obtained after saturation exposures of CO 2 at RT are shown in Fig. 2c . Analysis of the spectral composition with m / z values up to 50 reveals that CO 2 , CO and O were the dominant desorption products; no evidence for the presence of other species, for example, O 2 and derivatives of CO 2 , such as formic acid and formaldehyde [21] , was found. The intensities of the CO 2 and CO TPD signatures were calibrated using the corresponding sensitivity factors. The O-atom TPD signal was calibrated using the sensitivity factor for CO 2 and distinguished from the background H 2 O (the partial pressure of H 2 O in our apparatus is <1 × 10 −10 Pa). All spectra were broad and covered the temperature range from RT to 1,273 K, indicating the presence of several types of binding sites. In particular, the CO 2 , CO and O species started to desorb at about 350, 400 and 700 K, respectively. Desorption of CO 2 was completed at about 1,200 K. In contrast, the yield of both CO and O drastically increased at temperatures >1,200 K, and neither CO nor O was completely desorbed at 1,273 K. These data clearly demonstrate that, unlike in other oxides, the main desorption product here is CO. We note that the shape of the CO TPD spectrum ( Fig. 2c ) differs remarkably from that for CO 2 , and their yields differ by a factor of three. This observation rules out the possibility that the detected CO is produced by cracking desorbed CO 2 in the ionizer of the mass spectrometer. Hence, we conclude that the CO originates from the CO 2 pre-adsorbed at the C12A7: e − surface. In contrast, in the case of C12A7:O 2− , which contains no anionic electrons, the amount of desorbed CO 2 is <50% of that detected for the C12A7: e − , the TPD CO spectrum has a profile similar to that for CO 2 , and the magnification ratio of the CO spectrum is close to the pattern coefficient for fragmenting CO 2 by the ionizer of MSQ-400 (see Methods). Finally, we observed that the TPD yields and spectral profiles did not change after more than 20 cycles of CO 2 exposure followed by TPD measurements up to ~1,273 K. However, if the TPD procedure was terminated at 1,000 K, the CO yield decreased gradually from one TPD cycle to another. This result suggests that the surface sites responsible for CO generation do not fully recover at ≤1,000 K, which points to the crucial role of the oxygen-deficient, that is, electron-rich C12A7 surface. According to our calculations (see Methods for details), there are five types of CO 2 adsorbed on the C12A7: e − surface. 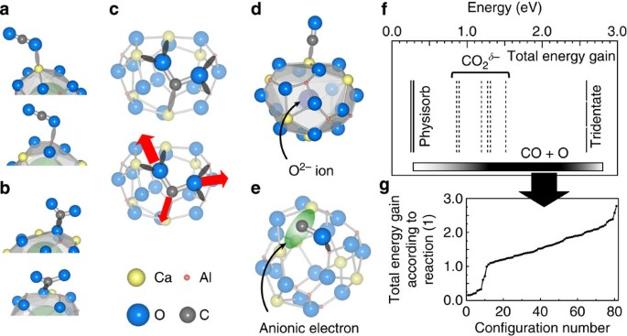Figure 3: Configurations and adsorption energies of CO2molecules adsorbed on C12A7:e−. (a–e) Geometrical configurations of a CO2molecule adsorbed on C12A7:e−surface: (a) physisorbed configuration, (b) CO2δ−, (c) tridentate CO2, (d,e) dissociation into O2−and CO species. (f) Adsorption energy ranges for the five types of CO2configurations: physisorbed CO2, bent CO2δ−, dissociated (two types) and tridentate. (g) Energy gain according to reaction (1) for all considered configurations of the resulting CO, including the bidentate CO and O2−. Figure 3 details their geometrical configurations and adsorption energies as calculated using the Perdew, Burke and Ernzerhof (PBE) density functional. Although the surface of C12A7: e − preserves the complex cage structure characteristic of bulk C12A7, it becomes partially disordered [22] . Therefore, each type of adsorbed CO 2 is characterized by a range of adsorption energies. The same applies to the reaction activation energies. The thermodynamically least stable species are physisorbed CO 2 (see Supplementary Note 1 ) having the calculated binding energy of about 0.3 eV (at least ~0.5 eV if the dispersion interaction is taken into account). In this case, the molecule binds to either a surface Ca or an Al atom and retains its linear configuration, as shown in Fig. 3a . Figure 3: Configurations and adsorption energies of CO 2 molecules adsorbed on C12A7: e − . ( a – e ) Geometrical configurations of a CO 2 molecule adsorbed on C12A7: e − surface: ( a ) physisorbed configuration, ( b ) CO 2 δ − , ( c ) tridentate CO 2 , ( d , e ) dissociation into O 2− and CO species. ( f ) Adsorption energy ranges for the five types of CO 2 configurations: physisorbed CO 2 , bent CO 2 δ − , dissociated (two types) and tridentate. ( g ) Energy gain according to reaction (1) for all considered configurations of the resulting CO, including the bidentate CO and O 2− . Full size image In more stable configurations, the C atom of CO 2 binds to a surface oxide ion, and the two C=O bonds are oriented away from the surface (see Fig. 3b ). This configuration is often referred to as bent CO 2 δ − , where δ is the amount of electron charge transferred from the C12A7: e − to the adsorbed, no longer linear, CO 2 molecule. The calculated adsorption energies for this configuration are 0.8–1.5 eV (1.2–2.3 eV in B3LYP), and the values of δ are 0.6–0.7 depending on the local atomic structure of the adsorption site. The ranges of C–O distances and O–C–O angles are 1.24–1.31 Å and 127–131°, respectively. The tridentate configuration, a special case of a bent and charged [23] adsorbed CO 2 molecule, is shown in Fig. 3c . Here the oxygen atoms bind to cations of a partially broken cage such that the molecule becomes part of the cage wall. The C–O distance elongates to 1.30 Å and the O–C–O angle decreases to ~117° so that the C atom faces one of the under-coordinated Ca 2+ ions. According to a Mulliken population analysis, over −1.6 | e | is transferred from the C12A7: e − to the molecule and is shared between the oxygen atoms and the central C atom, which forms a C–( e − )–Ca 2+ bond with a cage wall ion. The calculated adsorption energy for this configuration is 2.6 eV (4.5 eV in B3LYP) (see Supplementary Note 2 ). In addition, gas-phase CO 2 can be adsorbed via dissociation into O and CO species: where 0< k <2. In this reaction, two anionic electrons are transferred from the near-surface region to the O atom, which becomes an O 2− ion and occupies a site near the low-coordinated (LC) surface cations (M n+ ). The binding energy of the CO k − and the value of k depend on the local surface structure and the availability of anionic electrons. In particular, neutral CO molecules are physisorbed at the Ca 2+ ions with adsorption energies of up to 0.3 eV ( Fig. 3d ) and are chemisorbed forming OC–Al configurations with binding energies of up to 0.5 eV (>0.75 eV with the dispersion interaction) due to ~0.3 e transfer from C12A7: e − to the p -orbitals of the carbon atom. Alternatively, CO molecules bind between two or more LC surface cations forming ‘bidentate CO’ configurations ( Fig. 3e ) with binding energies in the range of 0.1–1.1 eV (0.7–2.2 eV in B3LYP). According to a Mulliken population analysis, as much as −1.5 | e | is transferred from the surface to the CO molecules. Hence, they are regarded as chemisorbed species, even though the binding energies can be small, and are represented as M 1 n+ —( e − )—CO − —M 2 m+ , where M 1 n+ and M 2 m+ are surface cations. The C–O bonds elongate to 1.27–1.34 Å depending on the details of the local atomic structure (see Supplementary Figs S1 and S2 ). We emphasize that the tridentate and dissociated O+CO configurations of CO 2 exist because of the unusual features of the C12A7: e − surface: (i) the partially broken cages that accommodate O atoms and the entire CO and CO 2 molecules and (ii) the high concentration and low binding energy of the anionic electrons, which stabilize the adsorbed O, CO and CO 2 . The adsorption energies calculated using the PBE functional increase by at least 0.15–0.2 eV when the dispersion interaction correction is applied [24] . CO 2 decomposition To test the feasibility of CO 2 →CO+O splitting (see reaction (1)), we considered several pathways, in which the resulting CO is physisorbed, and calculated the corresponding activation energies. For the physisorbed CO 2 , the lowest activation energy found is ~1 eV. Alternatively, the CO 2 pre-adsorbed at the surface in the bent CO 2 δ − configuration is split with an activation energy of ~1.5 eV. In all cases, one of the C=O bonds ruptures, and the oxygen atom traps two subsurface electrons and binds to LC cations as an O 2− ion. For the pathways that we have considered, this process is also accompanied by displacement of another surface O 2− ion into subsurface extra-framework sites via the interstitialcy diffusion mechanism that was found to dominate O 2− ion diffusion in bulk C12A7:O 2− (refs 25 , 26 , 27 ). The overall energy balance for reaction (1) is calculated as the sum of two contributions: (i) CO 2 →O+CO splitting in the gas phase followed by trapping the O atom at the surface according to O+2 e − →O 2− and (ii) adsorption of the CO molecule. The calculated energy gain for the former contribution is up to 1.7 eV (3.5 eV in B3LYP). Taking into account the adsorption energy for the bidentate CO, the total energy gain due to the dissociative CO 2 adsorption can be up to 2.8 eV (5.7 eV in B3LYP). This wide range of calculated CO 2 and CO adsorption energies correlates well with the broad multiple-peak TPD spectra. 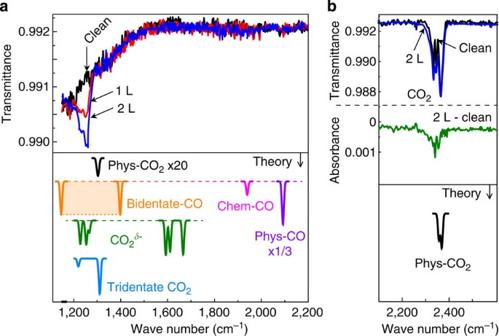Figure 4: FTIR-RAS spectra and wave number position of possible surface species. (a,b) FTIR-RAS spectra of the C12A7:e−surface after various (clean, 1 and 2 L) levels of exposure to CO2at RT. (b) Clean and 2 L spectra near the background gaseous CO2band and difference spectrum of them. Infrared spectroscopy Figure 4 shows FTIR-RAS spectra for a clean surface of C12A7: e − and one exposed to CO 2 gas at RT. Non-negligible infrared bands appear in the ranges of 1,200−1,280 and 2,300−2,400 cm −1 . The intensity of the 1,200−1,280 cm −1 band saturates after 2 L of CO 2 exposure, which is in good agreement with the TPD and PES (shown below) results, suggesting that this band originates from the adsorbed CO 2 . This band did not disappear until the sample temperature was raised >1,273 K. The 2,300–2,400 cm −1 band ( Fig. 4b ) overlaps with the background gaseous CO 2 band (BG). The intensity of BG randomly changed by the minute. Therefore, we evaluated the qualitative difference between spectra for the clean and one exposed to 2 L of CO 2 , which arbitrarily uniformed by the infrared band centred at 2,361 cm −1 derived from gaseous CO 2 . Here, the ‘2 L’ spectrum is expanded to normalize its intensity with the ‘clean’ spectrum. This procedure puts the maximum of the infrared band due to adsorbed CO 2 at 2,345 cm −1 . Figure 4: FTIR-RAS spectra and wave number position of possible surface species. ( a , b ) FTIR-RAS spectra of the C12A7: e − surface after various (clean, 1 and 2 L) levels of exposure to CO 2 at RT. ( b ) Clean and 2 L spectra near the background gaseous CO 2 band and difference spectrum of them. Full size image To assign these infrared features, we calculated the vibrational frequencies and infrared intensities for all types of adsorbed CO 2 . The physisorbed near-linear CO 2 was found to be the likely origin of the 2,300−2,400 cm −1 infrared band, as it has an infrared-active mode at ~2,360 cm −1 (asymmetric stretching) and an infrared-inactive mode at 1,300–1,315 cm −1 (symmetric stretching). In the CO 2 δ − configurations, the asymmetric and symmetric stretching modes transform into 1,660–1,680 and 1,210–1,260 cm −1 bands, respectively. Both bands are infrared-active and have comparable intensities. As the experimental data show no indication of infrared absorption in the 1,660–1,680 cm −1 range, we conclude that the CO 2 δ − configurations do not form in C12A7: e − at RT, which is consistent with the calculated formation energies of CO 2 δ − being smaller than those of the tridentate and dissociated O+CO configurations. However, this does not preclude the formation of transient CO 2 δ − species as, for example, precursors to O+CO configurations. Importantly, because the CO 2 δ− species, tridentate and O+CO configurations are stabilized by electron transfer from C12A7: e − , the concentration of these species is limited by the availability of such electrons in the near-surface region. In the case of the tridentate configuration ( Fig. 3c ), the two most active modes are similar to the asymmetric and symmetric vibrations of a water molecule and have calculated frequencies of ~1,310 and ~1,210 cm −1 , respectively, and an intensity ratio of approximately 4:1. As shown in the lower panel of Fig. 3c , the tridentate CO 2 molecule is effectively pulled apart by the oxygen atoms binding to two Ca 2+ ions on one side and one Al 3+ on the other and by the central C atom forming a C–( e − )–Ca 2+ bond with the cage wall. The calculated frequencies agree well with the experimental data, which explains the existence of two bands in the 1,200–1,300 cm −1 region with the lower-energy band having a lower intensity, and are consistent with the calculated high thermodynamic stability of the tridentate CO 2 . Finally, for the O+CO configurations, the calculated stretching frequencies for the bidentate CO are in the range of 1,150–1,410 cm −1 . Generalized gradient approximation (GGA) functionals are known to overdelocalize electronic defect states. In the case of M 1 n+ –( e − )–CO − –M 2 m+ configurations, this would result in an underestimated M 1 n+ –( e − )–C binding and, consequently, overestimated CO stretching frequency. Therefore, we conclude that the calculated infrared frequencies of the bidentate CO are consistent with the experimentally observed infrared absorption band at 1,200–1,300 cm −1 . The infrared signatures of the chemisorbed and physisorbed monodentate CO are at 1,900 and 2,100 cm −1 , respectively. Although the FTIR-RAS spectra show no noticeable infrared absorption in this frequency range, this does not preclude the existence of chemisorbed CO. Indeed, transfer of a fraction of an electron to the C atom of the adsorbed CO reduces its dipole moment and may result in infrared-silent CO species. Thus, comparison of these theoretical results with experimental infrared spectra suggests that tridentate CO 2 , bidentate CO, physisorbed CO 2 and, possibly, chemisorbed monodentate CO species co-exist at the C12A7: e − surface (see Table 1 ). We note that FTIR-RAS data alone are not sufficient to resolve between the tridentate CO 2 and bidentate CO configurations; hence, these results must be accompanied by other spectroscopic measurements. Table 1 Possible species adsorbed on C12A7: e − surface and their experimental observation. 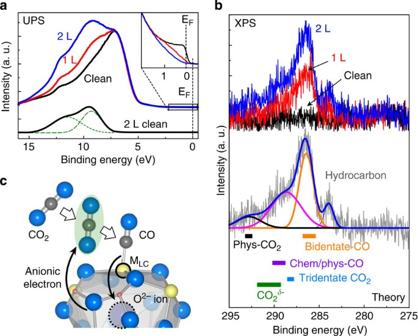Figure 5: PES spectra. UPS (He I) (a) and XPS (b) spectra of the C12A7:e−surface after various (clean, 1 and 2 L) exposures to CO2at RT. Inset inashows magnification of the spectra. Bottom ofbshows C 1senergy level of possible surface species: physisorbed CO2(phys-CO), bent CO2δ−, dissociated (two types) and tridentate CO2derived from calculation. Considering the FTIR results, the XPS signal could be assigned to bidentate CO (orange), phys-CO2(black), tridentate and possibly chemisorbed (chem) and phys-CO (pink) and hydrocarbon contaminants (grey). (c) Schematic illustration of dissociation of CO2(reaction (1)). The green-shaded spheres indicate transferred electronic charge from anionic electron to CO2. Full size table Photoelectron spectroscopy Figure 5a shows ultraviolet photoelectron spectroscopy (UPS) spectra for a clean C12A7: e − surface and a surface exposed to CO 2 (1 and 2 L) at RT. The clean surface shows a well-defined Fermi edge (inset in Fig. 5a ) firmly attributed to anionic electrons. The spectrum taken after 1 L of CO 2 exposure exhibits two additional peaks at binding energies of 9.2 and 11.5 eV. After dosing the surface with 2 L of CO 2 , the intensity of both peaks increased and reached saturation without an observable binding energy shift. At the same time, the Fermi edge disappeared, indicating that the anionic electrons were consumed in reactions with adsorbed CO 2 . Figure 5: PES spectra. UPS (He I) ( a ) and XPS ( b ) spectra of the C12A7: e − surface after various (clean, 1 and 2 L) exposures to CO 2 at RT. Inset in a shows magnification of the spectra. Bottom of b shows C 1 s energy level of possible surface species: physisorbed CO 2 (phys-CO), bent CO 2 δ − , dissociated (two types) and tridentate CO 2 derived from calculation. Considering the FTIR results, the XPS signal could be assigned to bidentate CO (orange), phys-CO 2 (black), tridentate and possibly chemisorbed (chem) and phys-CO (pink) and hydrocarbon contaminants (grey). ( c ) Schematic illustration of dissociation of CO 2 (reaction (1)). The green-shaded spheres indicate transferred electronic charge from anionic electron to CO 2 . Full size image The X-ray photoelectron spectroscopy (XPS) C 1 s spectra, together with the calculated C 1 s energy levels for physisorbed CO 2 , bent CO 2 δ − , tridentate CO 2 , chemisorbed and physisorbed CO and bidentate CO, are presented in Fig. 5b . The XPS spectra show three distinct peaks at binding energies of 286, 289 and 292 eV. The peak at 289 eV is broader than those at 286 and 292 eV. The ratio of these peak areas is about 4:4:1. The intensity of these signals correlates well with the CO 2 dosage, which strongly suggests that the signal is derived from adsorbed CO 2 . The peaks at 286 and 289 eV are apparent after 1 L of CO 2 exposure and increases in magnitude at higher doses; these peaks do not disappear until the sample temperature is raised >1,273 K. This behaviour is similar to that observed for the 1,200−1,280 cm −1 FTIR band, which was associated with both the tridentate CO 2 and bidentate CO configurations. Taking into account the TPD and FTIR data, comparison of the XPS spectrum and the calculated C 1 s energies ( Fig. 5b ) allows us to make the following assignments: the peak at ~286 eV is attributed to bidentate CO; the peak at ~289 eV—to the tridentate (multidentate) CO 2 configurations; and the peak at ~292 eV—to physisorbed CO 2 . Our calculations also show that the bent CO 2 δ − , chemisorbed and physisorbed CO can also contribute to the 289 eV peak. The broadening of the ~289 eV peak is attributed to non-equivalent broken surface cages that result in various multidentate CO 2 configurations and, possibly, chemisorbed and physisorbed CO. Subsurface extra-framework species The subsurface region of the C12A7 framework manifests itself in two aspects. First, earlier studies have shown that O 2− ions occupying extra-framework sites in the near-surface cages can be more stable than those occupying LC surface sites [28] . Taking into account that C12A7 is a fast conductor of oxide ions [25] , [26] , [27] , this suggests that O 2− formed in reaction (1) can diffuse into the bulk C12A7: e − , thus, making the original surface site available for a new reaction. Second, CO molecules are stabilized in the framework cages by either trapping two electrons or reacting with an extra-framework O 2− species with binding energies of 1.35 and 1.50 eV, respectively. The resulting structures and geometrical parameters (shown in Supplementary Fig. S3 ) are surprisingly similar to those for the surface bidentate CO and tridentate CO 2 ; hence, we extend the use of these terms to the bulk species. Moreover, the calculated vibrational frequencies are 1,251 cm −1 for the bidentate CO and 1,244 and 1,316 cm −1 for the tridentate CO 2 , that is, in close agreement with the experimental data. Finally, the binding energy for the C 1 s level in the tridentate CO 2 is ~1.4 eV smaller than that for the bidentate CO, which is consistent with the assignments made for the surface species ( Fig. 5 ). Thus, the spectroscopic characteristics of these subsurface CO-derived species are consistent with both IR and XPS measurements and ab initio calculations. Table 1 summarizes the experimental observation of possible chemical species adsorbed on the C12A7: e − surface. Our experiments and computational modelling complement each other and provide a consistent picture of CO 2 interaction with the C12A7: e − surface as follows. (1) The C12A7: e − surfaces retain the basic features of the complex C12A7: e − bulk structure: bulk-like and broken cages. The cages are occupied by anionic electrons, which serve as anchors capable of trapping gas-phase molecules, such as CO and CO 2 . As the surface is corrugated and partially amorphous, configurations of adsorbed molecules are described by a distribution of binding energies rather than by a single value. (2) CO 2 adsorption gives rise to five configuration types ( Fig. 3 ): physisorbed CO 2 , bent CO 2 δ − , tridentate and dissociated CO+O, where CO is either in the bidentate or chemisorbed configurations. In addition, the CO can be stabilized in the subsurface region by interacting with extra-framework electrons and O 2− ions and by forming bidentate CO and tridentate CO 2 in the bulk cages. The calculated activation energy for reaction (1) (see Fig. 5c ) is 1–1.5 eV. (3) As the surface temperature increases, physisorbed CO 2 and CO (bidentate or chemisorbed) become desorbed starting at 350 and 400 K, respectively. We propose that at temperatures >400 K, some of the desorbed CO 2 originates from the CO+O recombination. At temperatures >700 K, this recombination is suppressed by faster atomic vibrations, and the CO 2 desorption drops while O-atom desorption appears. (4) At temperatures >1,100 K, all of the physisorbed CO 2 and most of the CO have left the surface. However, decomposition of CO 2 molecules at deep traps, such as tridentate configurations, becomes possible, which leads to a steep rise in desorption of both CO and O species. In summary, we have demonstrated that C12A7: e − surfaces can adsorb CO 2 molecules and split them into CO molecules and O atoms at RT. According to the results of TPD measurements, molecular CO is the main desorption product. We propose that this desorption has a bimodal distribution. The CO molecules, formed at the surface due to CO 2 decomposition at LC metal sites, desorb at T >400 K. At T >1,100 K, CO 2 molecules adsorbed in the tridentate and similar configurations break up, thus forming another channel for desorption of CO and O species and replenishment of the sites available for CO 2 chemisorption and splitting. As the mechanisms for the processes proposed here require no highly reactive species, such as metallic alkali or alkaline earth metals, nor high- and/or low-temperature conditions, C12A7: e − is promising for practical applications in CO 2 activation and splitting. This work provides a foundation for further research that is necessary to enable C12A7: e − to function as a CO 2 -decomposition catalyst. Sample preparation We prepared the C12A7: e − surface samples as follows. A 1-inch [Ca 24 Al 28 O 64 ] 4+ (O 2− ) 2 (C12A7:O 2− ) (refs 29 , 30 , 31 ) ingot was grown by the Czochralski method and sliced along (110) planes into single-crystal 3 × 13 × 1 mm 3 wafers [32] . The extra-framework oxygen ions were replaced with anionic electrons by heating the wafers at 1,373 K for 24 h under a titanium vapour atmosphere in an evacuated (~10 −1 Pa) silica glass tube. The concentration of anionic electrons (2 × 10 21 cm −3 ), as determined from the optical absorption intensity at 2.8 eV, indicated that all of the extra-framework oxygen ions were removed in this process [33] . The samples were mirror polished mechanically with oil-based diamond powder slurries (9, 3 and 1 μm particle sizes) and alumina powder slurry (50 nm particle size). The C12A7: e − surface samples were then transferred to an ultrahigh vacuum (UHV) apparatus with a base pressure of under 3 × 10 −8 Pa and cleaned using Ar + ion sputtering (5 keV, 4.8 nA cm −2 from the 45° off-normal direction) followed by resistive heating at 1,273 K for 10 min. This treatment is necessary to obtain a C12A7: e − surface that retains the bulk cage structure, exhibits metallic conductivity and has a low work function [22] . After cooling to RT, the clean surface and electronic structure were examined using in situ XPS (Mg Kα) and UPS (He I). Exposure of the samples to CO 2 (99.999% purity) (C 18 O 2 in the TPDs) was carried out by backfilling in the UHV apparatus through a variable leak valve. The gas line was evacuated and heated to ensure that the specimens remained clean. The injection port for the CO 2 had a 1-mm opening size inside the apparatus and was located 5 mm away from the samples. A quadrupole mass spectrometer (ULVAC; MSQ-400) was used to monitor the partial pressure of the injection gas during exposure. The exposure was measured in units of Langmuirs (L: 1.33 × 10 −4 Pa s.). After the samples were exposed to CO 2 gas, the UHV chamber was evacuated immediately to a 3 × 10 −8 Pa base pressure before performing in situ TPD, PES (XPS and UPS) and FTIR-RAS measurements. Temperature-programmed desorption TPD spectra were taken in the 300–1,273 K temperature range at a constant heating rate of 0.5 K s −1 using an SQ-400. The sample temperature was controlled via resistive heating with a homemade computer-controlled power supply. The upper limit of the sample temperature was determined by reference to the melting point of the sample [34] , [35] . The conditions required to achieve saturation of CO 2 adsorption on C12A7: e − were determined by monitoring the pressure level in the UHV apparatus during the TPD measurements and the TPD yield as a function of CO 2 exposure. Photoelectron spectroscopy PES measurements were performed using a hemispherical analyser (Omicron) with a commercial non-monochromatic ultraviolet photon source (He I line: hν =21.2 eV, Δ E =0.1 eV) and an X-ray source (Mg Kα line: hν =1,253.6 eV, Δ E =1.0 eV). During UPS measurements, the He I beam strikes the sample surface at an angle of 45° to the surface normal and illuminates a spot approximately 2 mm in diameter. In XPS, X-ray photons hit the surface at an angle of 60° to the surface normal, illuminating a spot several millimetres in diameter. All PES spectra were taken at RT and displayed as a function of the electron-binding energy with respect to the Fermi level. Fourier transform infrared reflection absorption spectroscopy FTIR-RAS spectra were taken at RT with an FTIR spectrometer (Bruker; Tensor 27). The infrared source and infrared detector were placed on the outside of the UHV apparatus. The spectra were obtained as a ratio of the single-beam spectra with the CO 2 adsorbate and with the clean surface of the C12A7: e − . All spectra comprised 256 scans taken at a 4-cm −1 spectral resolution. The infrared light beam, extracted from the spectrometer, struck the sample surface at an angle of 85° to the surface normal through a CaF 2 window. After reflection of the light from the sample surface, it passed through an exit CaF 2 window and was collected and focused onto a mercury cadmium telluride infrared detector cooled using liquid nitrogen. All optical paths were isolated from ambient air and were filled with dry nitrogen. Theory Computational modelling was carried out using density functional theory, with the generalized gradient approximation functional of PBE [36] , unless stated otherwise, and the projected augmented waves method [37] implemented in the Vienna ab initio simulation package [38] . The plane-wave basis set cutoff was set to 500 eV. The C12A7: e − surface was modelled using a quasi-two-dimensional slab, in which one of the near-surface cages hosts two electrons, as described in detail elsewhere [28] . The surfaces exhibit a large number of structurally similar but not identical surface sites, including LC Ca 2+ and Al 3+ sites. The super-cell parameters in the x–y plane and in the direction perpendicular to the surface were fixed at 12 and 24 Å, respectively. As the near-surface region is partially disordered [38] , the calculations were carried out for the Γ point of the Brillouin zone only. Activation energies for the CO 2 -decomposition process were calculated using the nudged elastic band method and eight images. The infrared intensities for individual CO x species were calculated with respect to a common reference. The dispersion correction was calculated using a previously implemented method [24] . The configuration pre-optimized using the PBE functional was used to calculate the adsorption energies (reported for the chemisorbed configurations alongside the PBE results), the C 1 s core levels with the hybrid density functional B3LYP [39] , [40] , the CRYSTAL09 package [41] and all electron Gaussian-type contracted basis sets for Ca (5 s ,4 p ,1 d ), Al (4 s ,3 p ,1 d ), O (4 s ,3 p ,1 d ) and C (9 s ,3 p ,2 d ) http://www.crystal.unito.it/Basis_Sets/Ptable.html . The reasons for using the B3LYP density functionals and the correlation of the corresponding adsorption energies are presented in the Supplementary Fig. S4 . How to cite this article: Toda, Y. et al. Activation and splitting of carbon dioxide on the surface of an inorganic electride material. Nat. Commun. 4:2378 doi: 10.1038/ncomms3378 (2013).